From lab to life: how wearable devices can improve health equity 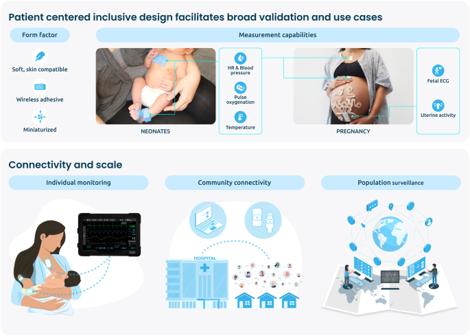Fig. 1: Application of advanced wearable devices for comprehensive monitoring of vulnerable patients at scale. Patient centered engineering and inclusive device design promote broad validation and various use cases. Deployment of low-profile sensors capable of comprehensive monitoring can encourage use in various vulnerable patient populations. Sensors can monitor an individual patient, producing physiological biomarkers for both personal and provider review in clinical and home environments. Low cost and reusable sensors facilitate scale. Further information on research design is available in the Nature Portfolio Reporting Summary linked to this article.